Broadband phonon mean free path contributions to thermal conductivity measured using frequency domain thermoreflectance Non-metallic crystalline materials conduct heat by the transport of quantized atomic lattice vibrations called phonons. Thermal conductivity depends on how far phonons travel between scattering events—their mean free paths. Due to the breadth of the phonon mean free path spectrum, nanostructuring materials can reduce thermal conductivity from bulk by scattering long mean free path phonons, whereas short mean free path phonons are unaffected. Here we use a breakdown in diffusive phonon transport generated by high-frequency surface temperature modulation to identify the mean free path-dependent contributions of phonons to thermal conductivity in crystalline and amorphous silicon. Our measurements probe a broad range of mean free paths in crystalline silicon spanning 0.3–8.0 μm at a temperature of 311 K and show that 40±5% of its thermal conductivity comes from phonons with mean free path >1 μm. In a 500 nm thick amorphous silicon film, despite atomic disorder, we identify propagating phonon-like modes that contribute >35±7% to thermal conductivity at a temperature of 306 K. Thermal conductivity ( k ), which relates the heat flux ( ) and temperature gradient ( T ) in a material through the Fourier law, , results from the cumulative contributions of phonons with a broad range of mean free paths (MFPs). The spectral MFP distribution is critical in nanostructured materials and devices, where size effects selectively scatter phonons or create non-Fourier conduction based on individual phonon MFPs. Such effects have an impact on heat dissipation in nanoelectronics and photonics, as well as the design of nanostructured thermoelectric materials with reduced thermal conductivity [1] , [2] , [3] , [4] , [5] , [6] , [7] , [8] , [9] . Because of its ubiquity in electronics, crystalline silicon (c-Si) has emerged as the prototypical material of study, yet controversy persists on what phonon MFPs dominate thermal transport, even in the bulk material. Kinetic theory defines the thermal conductivity as , where C is the volumetric heat capacity, v s is the speed of sound and Λ G is the average (or grey) MFP. For c-Si, kinetic theory yields Λ G =41 nm at a temperature ( T ) of 300 K [10] . This grey approximation severely underestimates the MFPs of the phonons that contribute significantly to thermal conductivity because (i) dispersion makes v s an overestimate of the average group velocity of acoustic phonons and (ii) optical phonons contribute to C but negligibly to bulk k (ref. 11 ). Thermal conductivity measurements of thin silicon films indicate that an effective MFP of 300 nm at T =300 K is more appropriate [12] . To clarify the spectral contributions of phonons to thermal conductivity as a function of MFP, Dames and Chen [13] established the thermal conductivity accumulation function, which identifies the thermal conductivity due to phonons having MFPs less than Λ*. To evaluate equation (1) analytically, models for phonon scattering must be chosen to form expressions for C (Λ) and v (Λ) [14] , [15] . There is no current consensus on how to select these models, which may be different for different materials. Furthermore, direct calculations of k accum at the phonon mode level by molecular dynamic simulations or lattice dynamics calculations [1] , [2] , [10] yield different behaviours for k accum than the analytical approaches. Discrepancies among predictions and a lack of information from conventional thermal conductivity measurements have motivated innovative experiments to probe phonon MFP spectra [1] , [16] , [17] , [18] , [19] , [20] . Koh and Cahill [16] found that the thermal conductivities of InGaP, InGaAs and SiGe alloys measured by time domain thermoreflectance (TDTR) depend on the surface heat flux modulation frequency ( f ). Periodic heat flux modulation induces an exponentially decaying temperature profile with a thermal penetration depth, , that identifies the depth normal to the surface at which the temperature amplitude is e −1 of its surface amplitude. Koh and Cahill reasoned that phonons with MFPs larger than L p travel ballistically and do not contribute to the measured thermal conductivity of the material (that is, TDTR measures k accum where Λ*= L p ). More recent inquiries to the MFP spectrum have set Λ* as the heat source dimension through the use of nano-patterned heaters on sapphire [17] , the TDTR spot-size on c-Si at cryogenic temperatures [1] and the grating period in transient grating experiments [18] , [19] , [20] . Spot-size limitations due to the diffraction limit of light and an upper limit to the modulation frequency achievable with pulsed lasers, however, restrict TDTR’s ability to probe a broad range of the MFP spectrum. Furthermore, the nano-patterning approach requires an optically transparent sample, whereas the transient grating observations of non-diffusive transport are as yet limited to thin membranes [19] , [20] . Hence, despite its intrigue, the MFP spectrum of bulk c-Si remains elusive at device operating temperatures. In this work, we apply broadband frequency domain thermoreflectance (BB-FDTR), a new technique, to measure phonon MFP spectra through variation of L p . The use of continuous wave (CW) lasers in BB-FDTR eliminates the multiple time scales associated with a pulsed-laser technique like TDTR [21] , [22] and, as we show in this work, enables fine resolution of an expanded range of L p . A schematic of BB-FDTR is shown in Fig. 1a . The 488 nm CW pump laser is intensity modulated by an electro-optic modulator and heats the sample surface at a frequency f 1 . The 532 nm CW probe laser senses the sample’s periodic temperature response based on the thermoreflectance of its surface. The phase-lag of temperature (probe) to heat flux (pump) is monitored by a lock-in amplifier. To vary L p and probe a wide range of MFPs, the pump beam is modulated from 200 kHz to 200 MHz. Increasing the frequency beyond 20 MHz causes signal-to-noise issues because the amplitude of the temperature response decreases, whereas coherent and ambient noise increase. To resolve this issue, we use a novel heterodyne approach (see Methods ). 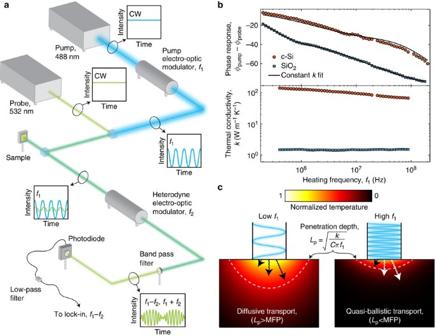Figure 1: BB-FDTR experiments reveal a heating frequency-dependent thermal conductivity. (a) Schematic of BB-FDTR technique used to measure phonon MFP spectra. (b) Phase-lag versus modulation frequency data for intrinsic c-Si and SiO2shown with a constant thermal conductivity fit over the entire experimental frequency range. Fitting SiO2yields a thermal conductivity value of 1.4±0.2 W m−1K−1, and window-fitting produces a heating frequency-independent thermal conductivity. Fitting c-Si over the entire frequency range yields a fitted thermal conductivity below bulk (99±6 W m−1K−1), and window-fitting shows a modulation frequency-dependent thermal conductivity. (c) Illustration of diffusive and ballistic transport. At low heating frequencies, when the thermal penetration depth is greater than the phonon MFPs, there is diffusive thermal transport, and a bulk value of thermal conductivity is measured. At high heating frequencies, the thermal penetration depth decreases below the MFPs of some phonons, which travel ballistically through the thermally affected zone (white arrows). These ballistic phonons do not contribute to the measured value of thermal conductivity. Figure 1: BB-FDTR experiments reveal a heating frequency-dependent thermal conductivity. ( a ) Schematic of BB-FDTR technique used to measure phonon MFP spectra. ( b ) Phase-lag versus modulation frequency data for intrinsic c-Si and SiO 2 shown with a constant thermal conductivity fit over the entire experimental frequency range. Fitting SiO 2 yields a thermal conductivity value of 1.4±0.2 W m −1 K −1 , and window-fitting produces a heating frequency-independent thermal conductivity. Fitting c-Si over the entire frequency range yields a fitted thermal conductivity below bulk (99±6 W m −1 K −1 ), and window-fitting shows a modulation frequency-dependent thermal conductivity. ( c ) Illustration of diffusive and ballistic transport. At low heating frequencies, when the thermal penetration depth is greater than the phonon MFPs, there is diffusive thermal transport, and a bulk value of thermal conductivity is measured. At high heating frequencies, the thermal penetration depth decreases below the MFPs of some phonons, which travel ballistically through the thermally affected zone (white arrows). These ballistic phonons do not contribute to the measured value of thermal conductivity. Full size image Heating frequency-dependent thermal conductivity Intrinsic c-Si (<1 × 10 12 cm −3 impurity atoms), doped c-Si (3 × 10 19 cm −3 boron atoms), amorphous SiO 2 (1 μm film thermally grown on c-Si), single crystal platinum (Pt) and amorphous silicon (a-Si) (500 nm, 1 μm and 2 μm films sputtered on c-Si) samples were sputtered with a Cr adhesion layer and a Au transducer (see Methods ). Au is our ideal transducer because it has high absorption at 488 nm (pump) and a high coefficient of thermoreflectance at 532 nm (probe) [23] . Phase-lag data from BB-FDTR is fit to an analytical solution of the diffusive heat conduction equation [21] . The unknown fitting parameters are the sample thermal conductivity and the Au-Cr/sample interface thermal conductance ( G ). Phase-lag versus modulation frequency data are shown in Fig. 1b for intrinsic c-Si ( T= 311 K) and SiO 2 ( T= 307 K). Also plotted are the best-fit lines when the entire frequency range is fit to a constant value of thermal conductivity. For SiO 2 , this fit yields a thermal conductivity of 1.4±0.2 W m −1 K −1 , which agrees with bulk values [24] and has a low mean square error (MSE=0.04). In intrinsic c-Si, however, the constant thermal conductivity fit underpredicts the bulk value (143 W m −1 K −1 (ref. 25 )) as 99±6 W m −1 K −1 with a large MSE of 2.4. Consequently, we divide the frequency range into overlapping windows of 13 points, and fit the thermal conductivity in each section (see Supplementary Methods and Supplementary Note 1 ). As shown in Fig. 1b , a frequency-dependent thermal conductivity is obtained. Window-fitting the phase data for SiO 2 , however, yields a frequency-independent thermal conductivity. In both cases, G is assumed to be frequency independent (see Methods ). Modelling the diffusive to ballistic transition To interpret the frequency dependence of the thermal conductivity measurements, the Boltzmann transport equation (BTE), which simultaneously considers diffusive and ballistic phonon transport, was solved using the lattice Boltzmann method (LBM) for an FDTR-like system (see Methods ) [11] , [26] . A modulated heat flux is applied to the surface of a large silicon medium, and the time evolution of the temperature within the entire domain is calculated. All phonons are assumed to have the same group velocity and MFP (that is, the grey approximation). From this data, we plot the steady-state temperature oscillation amplitude (Δ T ) as a function of sample depth for diffusive and ballistic transport regimes in Fig. 2a , Δ T at the surface (Δ T S ) as a function of L p in Fig. 2b and the perceived thermal conductivity based on Δ T S in Fig. 2c . The temperature amplitudes predicted by the Fourier law are plotted for comparison. At low heating frequencies, where L p >MFP, the BTE solution matches the Fourier prediction. As frequency increases and L p decreases, however, the BTE-predicted Δ T becomes larger than that predicted by the Fourier law, indicating an onset of ballistic phonon transport. In this case, phonons can travel ballistically through the thermally affected zone without scattering, as depicted in Fig. 1c . In the context of the BB-FDTR experiments, the BTE results should be interpreted as an observation of the transition of one phonon mode from diffusive to ballistic transport as the heating frequency is increased. Consistent with the BB-FDTR experiments, the BTE predicts a reduced thermal conductivity compared with bulk as the heating frequency is increased. 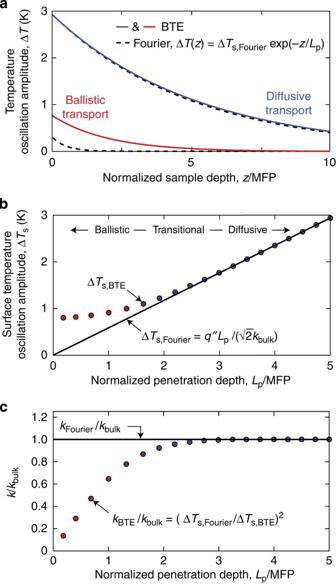Figure 2: BTEpredictions for the BB-FDTR experiment. (a) Spatial variation of the temperature oscillation amplitude for diffusive transport (corresponding to the lowest heating frequency inbandc) and ballistic transport (corresponding to the highest heating frequency inbandc) from the Fourier law (dashed line) and the LBM solution to the BTE for a grey material (solid line), all for a periodic surface heat flux. (b) Amplitude of the surface temperature oscillation and (c) perceived thermal conductivity plotted versus normalized penetration depth. WhenLp>MFP, the Fourier and BTE predictions match, and BB-FDTR experiments measure a bulk thermal conductivity. WhenLp<MFP, the Fourier law underpredicts the surface temperature oscillation amplitude, which is perceived as a reduced thermal conductivity, here and in BB-FDTR experiments. Figure 2: BTE predictions for the BB-FDTR experiment. ( a ) Spatial variation of the temperature oscillation amplitude for diffusive transport (corresponding to the lowest heating frequency in b and c ) and ballistic transport (corresponding to the highest heating frequency in b and c ) from the Fourier law (dashed line) and the LBM solution to the BTE for a grey material (solid line), all for a periodic surface heat flux. ( b ) Amplitude of the surface temperature oscillation and ( c ) perceived thermal conductivity plotted versus normalized penetration depth. When L p >MFP, the Fourier and BTE predictions match, and BB-FDTR experiments measure a bulk thermal conductivity. When L p <MFP, the Fourier law underpredicts the surface temperature oscillation amplitude, which is perceived as a reduced thermal conductivity, here and in BB-FDTR experiments. Full size image Experimental phonon MFP spectra By fitting our experimental data (which includes ballistic effects) with a purely diffusive model, we find an effective thermal conductivity. Our interpretation is that this effective thermal conductivity is k accum from equation (1), where only diffusive phonons that have MFP< L p contribute (that is, we are physically imposing Λ* =L p ). This interpretation is the same as that of Koh and Cahill [16] , and consistent with Minnich et al . [1] and Johnson et al . [19] , [20] who instead used the laser spot diameter and transient grating period as the cutoff dimensions. To generate a phonon MFP spectrum, the measured thermal conductivity at the median frequency of the i th fitting window ( f 1, i ) is plotted as a function of the corresponding penetration depth, (see Supplementary Methods ). Phonon MFP spectra for SiO 2 , intrinsic c-Si, doped c-Si, a-Si (500 nm film) and single crystal Pt near room temperature are compared in Fig. 3 . The thermal conductivities are normalized by their bulk values [24] , [25] , [27] , [28] , [29] . Shaded regions indicate uncertainty due to uncertainty in the thickness and thermal conductivity of the Au-Cr transducer, the laser spot-size, G , and the measured phase response (see Methods ). In SiO 2 , L p, i from 60–900 nm yield a constant value of thermal conductivity, which suggests that any phonon-like modes have a MFP spectrum that lies below 60 nm. The thermal conductivity of amorphous materials also has a contribution from non-propagating modes that have been called diffusons [30] . Because these modes do not propagate, there will be no observable transition between diffusive and ballistic transport as the BB-FDTR heating frequency is increased. This frequency-independent data is consistent with measurements of SiO 2 thin films where there was no observed thermal conductivity reduction from bulk due to boundary scattering [24] , [31] . In Pt, electrons with MFPs ~10 nm (ref. 32 ) are the dominant heat carriers, and strong electron–phonon coupling ensures that they are in thermal equilibrium with the lattice [33] . Thus, the thermal conductivity of Pt shows no L p dependence. 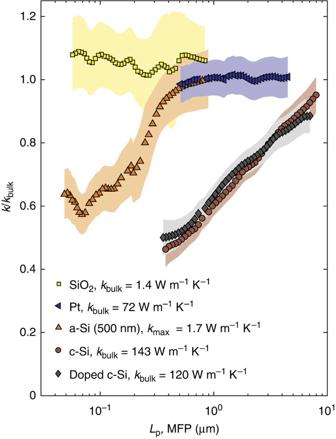Figure 3: Material-dependent phonon MFP spectra. MFP spectra for intrinsic c-Si, doped c-Si, a-Si (500 nm film), amorphous SiO2and Pt near room temperature. The thermal conductivity of SiO2is independent ofLp, suggesting that the MFPs of energy carriers are shorter than 60 nm. The MFP spectrum of Pt is independent ofLpbecause of short electron MFPs (~10 nm) and strong electron–phonon coupling in the metal. The MFP spectra of intrinsic c-Si and doped c-Si increase withLpand show that micron-long MFPs contribute significantly to bulk thermal conductivity atT=300 K. The MFP spectrum of the 500 nm a-Si film shows that propagating phonons with MFPs >100 nm contribute 35±7% to its thermal conductivity (for a-Si, we have used our maximum value for normalization). Figure 3: Material-dependent phonon MFP spectra. MFP spectra for intrinsic c-Si, doped c-Si, a-Si (500 nm film), amorphous SiO 2 and Pt near room temperature. The thermal conductivity of SiO 2 is independent of L p , suggesting that the MFPs of energy carriers are shorter than 60 nm. The MFP spectrum of Pt is independent of L p because of short electron MFPs (~10 nm) and strong electron–phonon coupling in the metal. The MFP spectra of intrinsic c-Si and doped c-Si increase with L p and show that micron-long MFPs contribute significantly to bulk thermal conductivity at T =300 K. The MFP spectrum of the 500 nm a-Si film shows that propagating phonons with MFPs >100 nm contribute 35±7% to its thermal conductivity (for a-Si, we have used our maximum value for normalization). Full size image In intrinsic c-Si, we probe L p from 0.3–8.0 μm and find that phonons with MFPs longer than 1 μm contribute 40±5% to the bulk thermal conductivity. We also note that 95±6% of the bulk thermal conductivity is obtained at the lowest heating frequency (200 kHz, L p ≈8 μm). This result underscores the importance of using low heating frequencies or steady-state measurements when attempting to measure bulk thermal conductivities. Relative to direct thermal conductivity measurements of c-Si thin films [12] and nanowires [8] , k accum at the film thickness or wire diameter is lower. In these nanostructures, phonons with MFPs greater than the limiting dimension are not excluded (as they are in BB-FDTR) and contribute to thermal conductivity with a MFP similar to the limiting dimension. Compared with intrinsic c-Si, the MFP spectrum of doped c-Si has a reduced slope, indicating that dopants broaden the MFP spectrum by adding an additional phonon scattering mechanism. Phonons scattered by dopants are forced to contribute to the thermal conductivity at a shorter MFP then they would in the intrinsic crystal. The nature of thermal transport in amorphous solids is a long-standing question in solid-state physics [34] . Often, as in our results for SiO 2 , the thermal conductivity can be described in terms of diffusons (that is, non-propagating modes). In contrast, our MFP spectrum for the 500 nm a-Si film shows that 35±7% of its bulk thermal conductivity comes from propagating (that is, phonon-like) modes with MFPs longer than 100 nm. Propagating phonon-like modes in a-Si were first inferred by a disagreement between thermal conductivity measurements and modelling predictions that was resolved by the consideration of low-frequency Debye modes [35] . More recent simulations and experiments have also pointed to the existence of long MFP phonon-like modes in a-Si [34] , [36] , [37] , [38] . Using atomistic calculations, He et al . [36] define modes with MFPs <10 nm as diffusons, which contribute approximately half to the bulk thermal conductivity. Phonon-like modes with MFPs >10 nm account for the remaining half. Our range of L p, i (40–1,000 nm) in a-Si accesses these phonon-like modes. The spectrum is flat below 100 nm as all of the propagating modes ballistically transmit through the domain, whereas the non-propagating modes remain diffusive. A steep transition occurs from 100–500 nm before the MFP spectrum asymptotes to a constant value as L p, i exceeds the film thickness (500 nm). Similar features exist in thicker films, though the transition is delayed to larger L p , indicating that k accum is influenced by the a-Si film boundaries (see Supplementary Discussion ). Phonon MFP spectra of intrinsic c-Si at temperatures of 81, 155, 311 and 417 K are shown in Fig. 4 normalized by bulk values [25] , [29] . The associated values of G , shown in the inset, are consistent with prior measurements of a Cr/Si interface [39] . At lower temperatures, longer MFP phonons contribute more significantly to the measured thermal conductivity. At temperatures of 81 and 155 K, the heat capacity is at 20 and 45% of saturation, respectively [40] . High-frequency phonon modes are not populated, and phonon–phonon scattering is reduced relative to T =311 K. At temperatures of 311 and 417 K, the population effects are less critical because the heat capacity is at 75 and 83% of saturation, respectively [40] . Instead, the shift in the MFP spectrum from T =311 K to T =417 K comes primarily from increased phonon–phonon scattering (that is, increased anharmonicity). 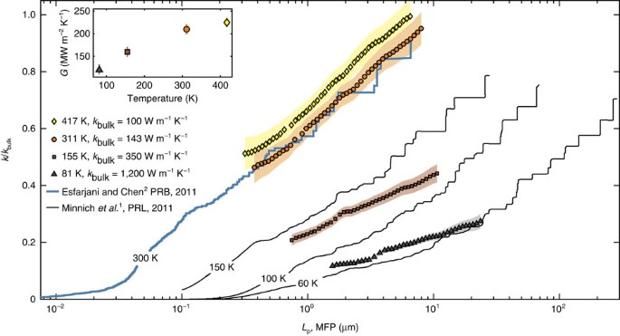Figure 4: Temperature-dependent phonon MFP spectra for c-Si. MFP spectra for intrinsic c-Si atT=81, 155, 311 and 417 K compared with MFP predictions from first principles calculations. Inset shows the temperature dependence of interface thermal conductance between the Au-Cr transducer and the intrinsic c-Si sample. The spectrum of phonon MFPs relevant to thermal conductivity shifts to lower values with increasing temperature due to increased phonon–phonon scattering. AtT=300 K, phonons with MFP>1 μm contribute 40±5% to bulk thermal conductivity. Comparison with predictions from Minnichet al.1and Esfarjani and Chen2are favourable at all temperatures. Figure 4: Temperature-dependent phonon MFP spectra for c-Si. MFP spectra for intrinsic c-Si at T =81, 155, 311 and 417 K compared with MFP predictions from first principles calculations. Inset shows the temperature dependence of interface thermal conductance between the Au-Cr transducer and the intrinsic c-Si sample. The spectrum of phonon MFPs relevant to thermal conductivity shifts to lower values with increasing temperature due to increased phonon–phonon scattering. At T =300 K, phonons with MFP>1 μm contribute 40±5% to bulk thermal conductivity. Comparison with predictions from Minnich et al . [1] and Esfarjani and Chen [2] are favourable at all temperatures. Full size image Although our data compare favourably with the first principles predictions by Esfarjani and coworkers [1] , [2] , [41] at all temperatures, one unresolved discrepancy is that a frequency-dependent thermal conductivity was not observed by TDTR experiments for c-Si at T= 300 K (ref. 16 ). Plausible explanations include (i) that a narrower frequency range (0.5–10 MHz compared with our range of 0.2–200 MHz) was considered, (ii) that the transducer material may affect the perceived frequency dependence (TDTR uses Al, whereas BB-FDTR uses Au-Cr) and (iii) that the radii of the laser beams, known to influence TDTR measurements of thermal conductivity at cryogenic temperatures [1] , was different (6.5–15 μm for TDTR relative to 3.4 μm for BB-FDTR). Our discovery that micron-long MFPs contribute substantially to k at room temperature and above suggests that silicon-based devices may have thermal management challenges in structures much larger than traditionally expected [10] , [12] . BB-FDTR’s continuous resolution of the MFP spectrum indicates how the dissipative ability of c-Si will continuously decrease as transistor size decreases to uphold Moore’s law. Likewise, BB-FDTR can aid in the understanding of thermal transport in amorphous solids by identifying propagating phonon modes and generating thermal conductivity accumulation functions. Our general experimental approach can be applied to measure the phonon MFP spectra of other semiconducting and insulating solids. Such bulk phonon MFP spectra can be extended to predict the thermal conductivity of thin films and nanostructures using the approaches of Yang and Dames [9] . Experimental details We use a novel heterodyne approach to reject ambient noise and coherent noise that are prohibitive to high-frequency measurements. A second electro-optic modulator induces an additional modulation on the probe beam at frequency f 2 after it is reflected from the sample surface (see Fig. 1a ). This method heterodynes the signal held by the probe beam into signals at frequencies of f 1 + f 2 and f 1 − f 2 . An optical band pass filter attenuates the pump beam so that only the probe beam reaches the photodiode. The photodiode output is passed through a low-pass electronic filter to reject the signal at f 1 + f 2 and is then connected to an SR-830 lock-in amplifier. We concurrently sweep f 1 and f 2 such that f 1 − f 2 is maintained at 86 kHz, which was chosen to minimize 1 /f noise without exceeding the low-pass cutoff of our filter. An electronic mixer is used to generate the reference for the lock-in amplifier at 86 kHz, and the phase-lag of the sample surface temperature with respect to the heat flux at f 1 are thus measured at 86 kHz. Our heterodyne approach enables robust high-frequency measurements limited only by the electro-optic modulator’s bandwidth. Phase-lag data are taken at 60 values of f 1 , evenly spaced on a log scale that spans 200 kHz to 200 MHz. For the frequency-dependent fits, the frequency range was broken into overlapping sections of 13 points, and G is determined by minimizing the MSE in the high-frequency range, where the phase response is most sensitive to its value (see Supplementary Methods ). A 1/ e 2 radius laser spot of 3.4±0.1 μm, measured using a knife-edge profiling technique, was used in this work (see Supplementary Methods ). Uncertainty, displayed as shaded regions in Figs 3 and 4 , was calculated using the procedure in Malen et al . [42] by considering uncertainty in the Au-Cr transducer thickness (±5%), the Au-Cr transducer thermal conductivity (±5%), G (sample dependant), spot radius (3.4±0.1 μm) and the propagation of error in the measured phase (see Supplementary Note 2 ). For SiO 2 and a-Si, a ±5% change in film thickness was also considered. Two assumptions are critical to the MFP spectra generated using this approach: (i) the transducer/sample interface thermal conductance is modulation frequency independent and (ii) the volumetric heat capacity is modulation frequency independent. Regarding (i), the relaxation time of electrons in Au is 3 × 10 −14 s at T =273 K (ref. 43 ). Because the time scale of our modulation frequency is minimally five orders of magnitude larger, the electrons and phonons will be in local equilibrium within the transducer over the entire modulation frequency range. Hence, the equilibrium of phonons and electrons at the interface is modulation frequency independent. Furthermore, this assumption is consistent with prior studies [1] , [16] . Regarding (ii), the long MFP phonons probed by BB-FDTR contribute substantially to thermal conductivity, but not to heat capacity (<1%) [2] . Sample preparation The transducer layer for all samples was prepared by depositing a ~5 nm Cr adhesion layer and ~55 nm of Au using a Perkin Elmer 6J sputtering system (see Supplementary Note 3 ). Before the sputtering process, the native oxide layers on intrinsic c-Si and doped c-Si samples were removed with a buffered hydrofluoric acid (HF) solution. The a-Si samples were sputtered on c-Si wafers in a low-pressure, argon-filled chamber. The c-Si wafers were first successively cleaned ultrasonically in acetone, isopropyl alcohol and deionized water and then submerged in a buffered HF solution to remove the native oxide layer. During the sputtering process, both the target and the wafer were cooled with recycling water. Low angle X-ray diffraction shows no crystalline peaks and confirms that the a-Si films are amorphous (see Supplementary Note S4 ). Profilometry was used to measure thicknesses of the a-Si films, and transducer layers were measured using X-ray reflectivity (see Supplementary Note S3 ). BTE solution methodology We use the LBM to discretize and solve the one-dimensional phonon BTE under the relaxation time approximation. The LBM provides the time and spatial dependence of phonon occupation numbers. From these phonon occupation numbers, temperature can be calculated using Bose–Einstein statistics. Details of our LBM methodology and numerical recipe are available in Nabovati et al (ref. 26 ). To use the LBM to solve the BTE for a BB-FDTR-like system, we consider a c-Si film under the grey approximation that is initially set to a uniform temperature of 300 K. The volumetric heat capacity is C =1.66 MJ m −3 K −1 , the speed of sound is v s =6,733 m s −1 and the bulk phonon MFP is Λ G =40 nm. Similar to the BB-FDTR experiment, a modulated heat flux of amplitude q′ and frequency f were applied at the free surface ( z =0). The heat flux modulation amplitude q′ is chosen such that the maximum surface temperature oscillation amplitude remains below 3 K for all frequencies. The boundary opposite to the heated surface is maintained at T =300 K. We choose sample thicknesses such that the propagating thermal wave decays to T =300 K well before it reaches the boundary opposite of the heated surface. We find that an 8 μm sample is sufficiently large for the penetration depths considered. We allow the system to evolve in time and report steady-state temperature oscillation amplitudes in Fig. 2a and surface temperature oscillation amplitudes in Fig. 2b . How to cite this article: Regner, K.T. et al . Broadband phonon mean free path contributions to thermal conductivity measured using frequency domain thermoreflectance. Nat. Commun. 4:1640 doi:10.1038/ncomms2630 (2013).